Efficient quantum state tomography Quantum state tomography—deducing quantum states from measured data—is the gold standard for verification and benchmarking of quantum devices. It has been realized in systems with few components, but for larger systems it becomes unfeasible because the number of measurements and the amount of computation required to process them grows exponentially in the system size. Here, we present two tomography schemes that scale much more favourably than direct tomography with system size. One of them requires unitary operations on a constant number of subsystems, whereas the other requires only local measurements together with more elaborate post-processing. Both rely only on a linear number of experimental operations and post-processing that is polynomial in the system size. These schemes can be applied to a wide range of quantum states, in particular those that are well approximated by matrix product states. The accuracy of the reconstructed states can be rigorously certified without any a priori assumptions. One of the principal features distinguishing classical systems from quantum many-body systems is that quantum systems require exponentially many parameters in the system size to fully specify the state, compared with only linearly many for classical systems. Put to use constructively, the exponential complexity enables the construction of information processing devices fundamentally superior to any classical device. At the same time, however, this 'curse of dimensionality' makes engineering tasks—such as verifying that the quantum processing device functions as intended—a daunting challenge. The full determination of the quantum state of a system, known as quantum state tomography [1] , has already been achieved by measuring a complete set of observables whose expectation values determine the quantum state [2] , [3] , [4] , [5] , [6] , [7] . As it is typically formulated [8] , simply to output an estimate for a generic state would take exponential time in the system size N , given that there are an exponential number of coefficients in a generic state's description. This is but one of several inefficiencies. Most quantum states have exponentially small amplitudes in almost every basis, so to distinguish any one of those amplitudes from zero, one must take an exponential number of samples. Assuming one were able to collect all the data from an informationally complete measurement, one is left with the intractable computational task of inverting the measured frequencies to find an estimate of the state. However, the traditional representation of quantum states is in a sense too general. Indeed, states that occur in many practical situations are specified by a small number of parameters. An efficient description could be a practical preparation scheme that outputs the state or, in the case of thermodynamical equilibrium states, a local Hamiltonian and temperature. This insight is not new: researchers in many-body physics and quantum information theory have found many classes of states, which are described by a number of parameters scaling polynomially in N [9] , [10] , [11] , [12] , [13] 9–13 and closely approximate the kind of states found in physical systems [14] , [15] . However, the question of whether these restricted classes can be put to use in the context of tomography has remained largely open. In this work, we address the above challenge. The physical system we have in mind is one where the constituents are arranged in a one-dimensional configuration (for example, ions in a linear trap [3] ). But the methods that we are presenting here can be generalized to higher-dimensional arrangements, such as those realized in optical lattices [16] . It is highly plausible that in such a setting, correlations between neighbouring particles are much more pronounced (due to direct interaction) than correlations between distant systems (mediated, for example, by global fluctuations of control fields). An efficiently describable class of states anticipating exactly this behaviour has long been studied under the names of finitely correlated states (FCS) or matrix product states (MPS) [9] , [10] . Importantly, restricting to this class is not a limitation as every state may be written as an MPS with a suitable, albeit possibly large, matrix dimension. As many states that are relevant for quantum information processing or quantum many-body physics have a small (independent of N ) bond dimension, our methods are directly applicable to such states; examples include, but are not limited to, ground and thermal states, the GHZ, W, cluster and AKLT states, the latter two being universal resource states for quantum computing. Here, we present two schemes for identifying systems that are well approximated by an MPS, initially focusing on pure states for simplicity. We will view each system as consisting of a linear chain of N particles (or qudits ), each having d internal degrees of freedom. Both schemes require the measurement of linearly (in the system size N ) many local observables within finite accuracy, as well as polynomial classical post-processing of the data. They can also certify the accuracy of the reconstructed state without making any technical assumptions about the state in the laboratory. The first scheme requires unitary control and local measurements, whereas the second scheme removes the need for unitary control at the cost of more elaborate post-processing. Given that standard tomography is no longer feasible in a range of recent and upcoming experiments involving large numbers of qubits, our results represent a significant advance in the ability to verify and quantitatively and efficiently benchmark systems of experimental importance. Scheme based on unitary transformations The key idea of the method consists of a sequential procedure to disentangle the left hand side of the chain from the right hand side, using a sequence of unitary operations with small interaction length independent of N . The result will be a product state and a sequence of local unitary operations from which to construct the original state. Suppose the ideal state in the laboratory is , which we assume for clarity is an MPS of given bond dimension. This implies that the rank of reductions to one part of a bipartite (left versus right) split of the chain is bounded by a constant R . The protocol starts by estimating, through standard state tomography, the reduced density matrix of the first κ = ⌈ ⌈ log d ( R ) ⌉ +1 sites, . This reduced density matrix has the eigendecomposition , where the rank R ≤ d κ−1 . Hence, there exists a density matrix with one fewer qudit that has the same rank R and eigenvalues σ r as . Therefore, we can disentangle the first site in with the following unitary acting on the first κ-sites: where | φ 1 〉,...,| φ R 〉 have been extended in some arbitrary way to get a complete basis for sites 1,..., κ . Applying Û produces the state , where | v 〉 is some pure state on sites 2,..., N . Hence, Û disentangles the first qudit from all the others. 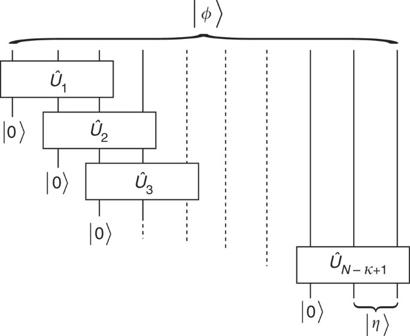Figure 1: Quantum circuit to obtain matrix product state. The circuit transforms. The unitariesÛisuccessively disentangle the particles and the state |η〉 on the last sites acts as a boundary condition to determine the MPS description of |φ〉. Now, set aside this first qudit, look at sites 2,..., κ +1, and repeat the above process as indicated in Figure 1 . In this way, one obtains a sequence of unitaries , where each Û i acts on sites i ,..., i + κ −1. This sequence transforms | φ 〉 into , where | η 〉 is some pure state on the last κ −1 sites. Figure 1: Quantum circuit to obtain matrix product state. The circuit transforms . The unitaries Û i successively disentangle the particles and the state | η 〉 on the last sites acts as a boundary condition to determine the MPS description of | φ 〉. Full size image In summary, this scheme infers the quantum circuit used to prepare an MPS [17] . The MPS decomposition of | φ 〉 can then be obtained readily from the U i and | η 〉 [18] . If the state in the laboratory ρ̂ is arbitrary, then the reduced density matrices will generally have full rank. Hence, in each step we will need to truncate the κ qudit state to a rank R subspace with R < d κ−1 . Then the above method will produce an MPS approximation to ρ̂ . The accuracy of this estimate can be certified, without any assumptions on the state, by keeping track of the effects of truncating each of the reduced states . As shown in the Methods, errors of magnitude ɛ due to finite measurement precision or truncation error (as measured by the weight of the truncated space) accumulate at most linearly with the number of sites, and can be evaluated directly from the data, leading to an estimate of accuracy N ɛ. The present scheme requires unitary control of κ neighbouring qudits, which is challenging to implement in many current experimental settings. We now present a second scheme that avoids unitary control and requires only local measurements. Certification of the estimated state Consider again the state ρ̂ in the laboratory and suppose that a tomographically-complete set of local measurements on all groups of k neighbouring qudits has been performed. Further suppose that sufficient data has been taken to yield estimates of the local reductions such that Determining these approximate reduced density operators completes the experimental work. In the remainder we describe the classical post-processing that will result in an MPS estimate | ψ 〉 to ρ̂ and a lower bound to the fidelity [19] that does not require assumptions on the nature of the state ρ̂ . We start with the latter, as the following easy calculation yields the fidelity bound we have in mind and hints at the MPS estimate we are after. Suppose, for the sake of the argument that | ψ 〉 is the unique ground state (with energy zero) of a local Hamiltonian , where the is a projection operator acting only on sites i +1, ..., i + k (as it turns out, generic MPS are of this type). Then, expanding in the eigenbasis , where we denoted by Δ E the energy gap above the ground state | ψ 〉. Hence, we have the fidelity bound In other words, the Hamiltonian acts as a witness for its ground state | ψ 〉. This bound is tight: suppose the experimental estimates and the reductions of the state in the laboratory ρ̂ i coincide, that is, ɛ i =0. If, in addition, the reductions of | ψ 〉 match the then, as | ψ 〉 was assumed to be the unique ground state with energy zero of , we have , that is, . The goal is now clear: find a local gapped Hamiltonian Ĥ such that the reductions of its ground state are close to the . A priori it is unclear whether such a convenient witness always exists and how it could be found efficiently. However, using formal methods, one can show that if the true state ρ̂ is close to a generic MPS, then such a witness Hamiltonian always exists [10] if we chose . What is more, it can be constructed from the estimate of the algorithm sketched below. Its properties, chief among them the gap, are efficiently computable. In the Methods section, we detail the efficient computation of these quantities, and we also consider how to treat states, such as the GHZ, for which local marginals alone are not quite sufficient for complete characterization (they violate our 'generic' condition). An illustrative example We illustrate how our certification procedure operates if our estimate for the state ρ̂ is a linear cluster state [20] . The cluster state is defined as the unique eigenstate (with eigenvalue +1) of stabilizers for all (together with boundary terms and , which we do not treat separately for simplicity). Assume that we have performed standard quantum state tomography on sets of three neighbouring spins, k =3, which is the smallest useful set because in a cluster state the rank of the reduced density matrices of contiguous blocks is upper bounded by R =4. Let us now assume that on the basis of these data, our procedure suggests that the linear cluster state is indeed our estimate. The local Hamiltonian in this case is given by , where the are projectors, Ĥ has the cluster state as its unique ground state (with energy zero) and an energy gap Δ E =1. The fidelity between the cluster state | ψ CS 〉 and the state ρ̂ is bounded by , where ɛ i from equation (3) quantifies the statistical and experimental error in the local experimental estimates, and quantifies how much the laboratory state ρ̂ deviates from an exact cluster state. Tomography on a cluster state can also be performed with the scheme based on unitary transformations. A cluster state is the output of a quantum circuit where each qubit is initially prepared in the state and a controlled phase transformation CZ acts successfully on each pair of neighbouring qubits. The CZ gate changes the sign of state |11〉 and acts trivially on the other states of the computational basis. Thus, a cluster state is the output of a circuit whose structure corresponds to the one indicated in Figure 1 , with κ =2 and the scheme based on unitary transformations directly applies. Note that the unitary scheme takes advantage of the decreased rank of a reduced density matrix on the boundary to save one qubit worth of local tomographic effort ( κ =2 versus κ =3). Efficient determination of an MPS estimate With the experimentally obtained we now turn to the task of finding an MPS | ψ 〉 such that its reductions closely match the . In other words: Let be all possible products of Pauli operators (enumerated by m ) that act non-trivially only on sites i +1 ,..., i + k . Then, as the are an orthogonal basis, the may be expanded as where the expectations are obtained as results of tomographic measurements. Then we need to find a matrix , such that for all m and i the expectations coincide with those of the tomographic estimates, . The method of choice for such a problem is singular value thresholding (SVT) [21] , [22] , which has been developed very recently in the context of classical compressive sampling or matrix completion [23] and may also be applied to the quantum setting [24] , [25] , [26] , [27] , [28] . SVT is a recursive algorithm that provably converges to a low-rank matrix satisfying constraints of the type . Unfortunately, a straightforward application of SVT requires time and memory that scale exponentially with the number of particles. However, a modification of the algorithm allows us to overcome this problem. Given the measured values the algorithm may then be described as follows. First, set up the operator and initialize to some arbitrary matrix (for example, the zero matrix). Then proceed recursively by finding the eigenstate | y n 〉 with largest eigenvalue, y n , of and set So far, this algorithm still suffers from the fact that in every step the 2 N ×2 N matrix needs to be diagonalized. However, the are of the form , where the act non-trivially only on sites i +1, ..., i + k , that is, they have the form of a local 'Hamiltonian'. Hence, | y n 〉 can be determined as the highest energy state of this Hamiltonian. For this task, standard methods have been developed in condensed matter physics [13] , [29] , for which the number of parameters scale polynomially in the system size and converge rapidly [30] , [31] to the optimal MPS approximation. The standard but exponentially inefficient SVT algorithm possesses a convergence proof, whereas our efficient modification does not. Hence, we now present numerical examples for different target states | φ 〉 to demonstrate the feasibility and efficiency of the proposed algorithm. These numerical examples suggest convergence of our algorithm to an MPS that closely matches the experimentally obtained reductions . To arrive at the fidelity bound, we follow the steps of Section 'Certification of the estimated state': (1) Obtain estimates of the reductions to k adjacent spins ρ̂ i of the state in the laboratory such that , (2) compute the expectations , which are the input to the MPS-SVT algorithm, (3) obtain an MPS estimate | y n 〉, the reductions of which closely match the by utilizing the MPS–SVT algorithm. As | y n 〉 is an MPS, one can then efficiently obtain a parent Hamiltonian [10] and a lower bound, Δ, on the energy gap above the ground state (see Methods for details). Putting all this together, the above programme returns a state | y n 〉, its parent Hamiltonian , and a number Δ such that Strongly interacting quantum systems example We start with ground states of nearest-neighbour Hamiltonians on a chain, that is, the | φ 〉=| gs 〉 are completely determined by all the reductions to two adjacent spins and we expect the above algorithm not only to produce states that match the reduced density matrices of the ground states but, in fact, also states that are themselves close to the ground states. Among ground states of one-dimensional nearest-neighbour Hamiltonians, those at a critical point are the most challenging to approximate by MPS as they violate the entanglement area law [32] . We demonstrate the effectiveness of our algorithm for such an example: the critical Ising model in a transverse field on a chain of length N with open boundary conditions. The ground state of this Hamiltonian is unique and hence it is completely characterized by its reductions to k =2 neighbouring sites. In other words, if we find an MPS that has the same reductions, the fidelity will be one. We proceed as follows. (1) We obtain the reductions ρ̂ i to two neighbouring sites of the true ground state, (2) from these reductions we obtain the expectations , which are the input to the MPS-SVT algorithm. 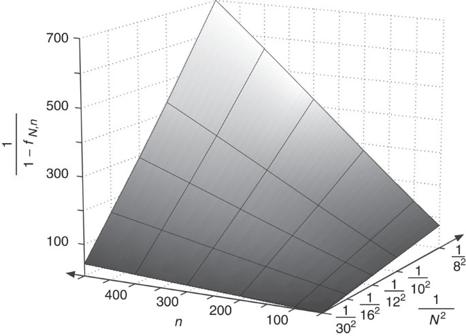Figure 2: Performance of the MPS–SVT algorithm for the ground state of the critical Ising model. We chosek=2, that is, only nearest-neighbour reductions are used to reconstruct the state. Plot illustrates the scaling of the error in the fidelitywith the number of spinsNand the iterationsnof the algorithm. In Figure 2 , we show the fidelity f N,n =|〈 y n | φ 〉| 2 of the true ground state | φ 〉 and the n 'th iterate of the above algorithm as a function of n and the length N of the chain. It shows that for fixed system size 1− f N,n decreases as ∼ 1/ n , whereas for fixed n it increases slower than N 2 . This provides an indication that our algorithm is polynomial in the system size. Figure 2: Performance of the MPS–SVT algorithm for the ground state of the critical Ising model. We chose k =2, that is, only nearest-neighbour reductions are used to reconstruct the state. Plot illustrates the scaling of the error in the fidelity with the number of spins N and the iterations n of the algorithm. Full size image The Ising model is solvable and, in order to show that we are not considering a special case that is particularly favourable, we also consider one-dimensional random Hamiltonians of the form where the act on spin i and i +1, respectively, and are hermitian matrices with entries that have real and imaginary part picked from a uniform distribution over [−1,1]. 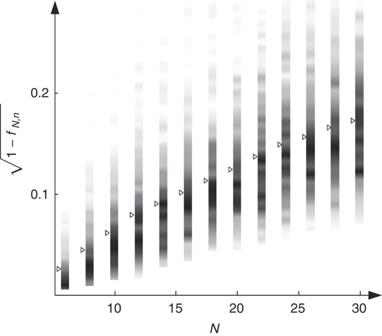Figure 3: Performance of the MPS–SVT algorithm for ground states of random Hamiltonians. FidelityfN,n=|〈φ|yn〉|2, for a fixed valuen=5, as a function of the number of spinsNfor the ground state (the target state |φ〉) of the random nearest-neighbour Hamiltonians of equation (8). As inFigure 2, we chosek=2 to reconstruct the state. The plot shows densities (arrows indicate the mean) obtained from 1,000 random realizations. Similar to the Ising model, the scaling for fixednof 1−fN,nis better than∼N2. For each Hamiltonian, as before, we first determine the ground state | gs 〉 (our target state | φ 〉) and its reductions and then computed the fidelity f N,n after n iterations of the MPS–SVT algorithm, see Figure 3 . Figure 3: Performance of the MPS–SVT algorithm for ground states of random Hamiltonians. Fidelity f N,n =|〈 φ|y n 〉| 2 , for a fixed value n =5, as a function of the number of spins N for the ground state (the target state | φ 〉) of the random nearest-neighbour Hamiltonians of equation (8). As in Figure 2 , we chose k =2 to reconstruct the state. The plot shows densities (arrows indicate the mean) obtained from 1,000 random realizations. Similar to the Ising model, the scaling for fixed n of 1− f N,n is better than ∼ N 2 . Full size image W-state preparation in ion traps Our method is of interest for many situations, in which standard tomography will not be feasible. This is the case for the verification of state preparation in experiments with too many particles. An example is the recent ion trap experiment [3] for the preparation of W-states, , that were limited to 8 qubits principally because the classical post-processing of data became prohibitive for longer chains. Here, we demonstrate the efficiency of our approach (we are not limited to few ions and demonstrate convergence for up to 20 ions—even higher number of ions are easily accessible due to the MPS alteration of the SVT method) by illustrating how one would post-process experimentally obtained reduced density matrices to guarantee the generation of | φ 〉 or a state very close to it. Note that, as in the above spin chain examples, one need only take tomographic data on pairs ( k =2) of neighbouring qubits. We mimic experimental noise by adding Gaussian distributed random numbers with zero mean to the . After initializing the algorithm with , where we obtain from the MPS representation of | φ 〉, we use as a figure of merit for convergence, that is, after a given number of iterations, we pick the | y n 〉 with minimum x n . 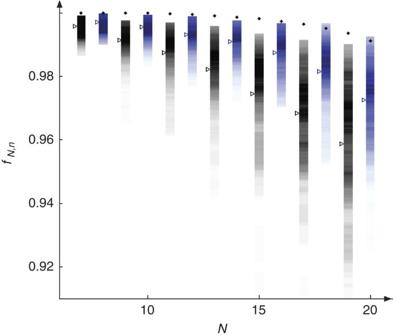Figure 4: Performance of the MPS–SVT algorithm for W-states. We are not limited to few ions and demonstrate convergence for up to 20 ions—even higher number of ions are easily accessible due to the MPS alteration of the SVT method, demonstrating the efficiency of our approach. We mimic experimental noise by adding Gaussian distributed random numbers with zero mean to the local expectationsand show results forn=4,000 MPS–SVT iterations. Plot showsfN,n=|〈φ|yn〉|2as a function of the number of ions,N, for no noise (dots) and Gaussian noise (densities obtained from 100 realizations for eachN, arrows indicate mean) with a s.d. 0.005 (blue; only even values ofNplotted for clarity) and 0.01 (black, oddN). The result of such a procedure is shown in Figure 4 . Figure 4: Performance of the MPS–SVT algorithm for W-states. We are not limited to few ions and demonstrate convergence for up to 20 ions—even higher number of ions are easily accessible due to the MPS alteration of the SVT method, demonstrating the efficiency of our approach. We mimic experimental noise by adding Gaussian distributed random numbers with zero mean to the local expectations and show results for n =4,000 MPS–SVT iterations. Plot shows f N,n =|〈 φ|y n 〉| 2 as a function of the number of ions, N , for no noise (dots) and Gaussian noise (densities obtained from 100 realizations for each N , arrows indicate mean) with a s.d. 0.005 (blue; only even values of N plotted for clarity) and 0.01 (black, odd N ). Full size image We have presented two schemes that efficiently produce an MPS description as a tomographic estimate of a quantum state, along with a tight fidelity bound. We emphasize that no assumptions are necessary for our scheme; if no such MPS description exists, this will be evident from the local tomographic data and our schemes will herald a failure. However, the enormous successes of MPS for describing both one-dimensional quantum systems found in nature as well as a host of states relevant to quantum information ensures that our methods will be very useful in practice. So far we presented the method for pure states and one-dimensional systems. Various generalizations are possible: Our first scheme using unitary control can also handle mixed states corresponding to small ensembles of pure MPS. Suppose we are presented with a state ρ̂ that is a mixture of M -pure states, each of which is an MPS having bond dimension D . Then the reduction of ρ̂ to any subsystem has rank at most MD . We can proceed as before, performing unitary operations on blocks of κ = ⌈ log d (MD) ⌉ +1 sites, to disentangle individual sites from the rest of the chain. At the end of the chain, we will find a mixed state η of rank M on the last κ −1 sites. We decompose η as a mixture of M -pure states. This yields a representation of ρ̂ as an ensemble of M -pure MPS, each with bond dimension at most dMD . Our second scheme using local measurements can also be extended to handle mixed states. While the k -particle reduced density matrices do not uniquely determine the mixed state ρ̂ , reconstructions of better and better quality can be obtained by increasing k . As an example, suppose ρ̂ is the Gibbs state corresponding to a k -local Hamiltonian Ĥ , that is, the state minimizing the free energy The first term is, as before, determined by the reduced density matrices. The entropy of the total state, however, can only be learned exactly from the complete density matrix. Yet, for essentially all reasonable physical systems, the entropy density in the thermal state of a Hamiltonian exists [33] (In particular, FCS are precisely those states whose entropy density is exactly equal to for some finite value of k ). As a consequence, the total entropy of the state can be estimated efficiently from knowledge of the reduced density matrices. Hence, our second scheme using local measurements may be extended to mixed states by considering purifications and can then, for example, also handle thermal states of local Hamiltonians, under the physically reasonable assumption that the entropy density exists [33] . In addition, it can be generalized to all mixed FCS [9] , though it is not always possible to certify the resulting estimates. Higher-dimensional systems are more challenging, because the most straightforward generalization of MPS, known as projected entangled-pair states [34] , cannot be computed as efficiently. However, the certification method using a frustration-free parent Hamiltonian remains efficient in the case of qubits with nearest-neighbour couplings [35] . Combinations of our techniques can be used to reconstruct other classes of states, such as tree tensor networks [36] and multiscale entanglement renormalization ansatz states [37] , for which efficient heuristics for minimizing local Hamiltonians are available. Matrix product states We start by recalling the MPS representation of a state | ψ 〉 with open boundary conditions (generalizations to periodic boundary conditions are entirely straightforward). ,where the M i [ s ] are D i = × D i +1 matrices with D 1 = D N +1 =1. We denote the bond dimension by D =max D i . Direct tomography This method proceeds by disentangling all the qudits of the chain sequentially. Thus, it yields a valid MPS description if every unitary exactly disentangles one qudit. Put another way, while it is crucial to obtain a good estimate of the d κ −1 -dimensional subspace on which is supported, it is not necessary to identify the eigenvectors of exactly: any set of orthonormal vectors generating the subspace is sufficient for our tomography procedure and leads to an MPS description in another gauge [10] . This property will be central to our error analysis. To understand the effect of errors and imperfections in our tomography procedure, consider the very first step of the recursive procedure. Tomography is performed on the first κ -sites to ideally find a state with non-maximal support, and unitary is applied to rotate that state into the subspace . In any experimental setting, the resulting state would surely not lie entirely in that subspace. This can be either because the state of the system is not exactly an MPS with bond dimension D , but merely close to one or because our estimate of the density matrix on sites 1 to κ is slightly wrong due to measurements that are, in practice, noisy and restricted to finite precision. Indeed, we can expect that the reduced density matrix on the first κ-sites will actually be full-rank, although most of its probability mass will lie on a subspace of dimension at most D. So, each time we apply a disentangling operation , we also want to truncate the reduced state to the desired subspace. Similarly, a faulty estimate of will result in a small probability mass that lies outside the estimated support. Given an estimated disentangling unitary , any state | φ 〉 can be expressed as ,where | e 1 〉 is some subnormalized error vector supported on the subspace orthogonal to . The unitary is chosen to minimize the norm ɛ 1 = 1 | e 1〉 of this error vector. It is possible to directly estimate the magnitude of the error ɛ 1 by measuring the first qudit in the standard basis; the error is equal to the population of the non-zero states. In subsequent steps of the recursion, we are given a state of the form ,where is the accumulated error vector that lies in the subspace orthogonal to . As a first step, we can truncate this error vector by measuring the first i particles in the standard basis and post-select on the all-zero outcome. This occurs with a probability roughly , and leaves the system in the state . We then repeat the steps leading to equation (11) with the post-selected state . The resulting state will be where and therefore . Thus, we see that errors accumulate linearly with the number of particles; if we denote the estimated MPS, we have where ɛ =max i ||| e i 〉||. The overall error is at most the sum of the individual errors on each step. In addition, each of the ɛ i is revealed during the tomographic procedure because they correspond to the post-selection success probability. This provides a direct method to certify the inferred state. Parent Hamiltonians Let | ψ 〉 be as in (10) and such that for all i =1,..., N . This can always be achieved by subsuming qudits at the beginning and end of the chain into qudits with higher dimension and successive singular value decompositions [9] , [10] . Now let N , k ∈ N such that N / k ∈ N , and assume that the MPS is injective [10] such that for all j = k , ..., N –2 k the set spans . Then | ψ 〉 is the unique ground state of where is the projector onto the subspace orthogonal to the range of the mapping , To get an efficiently computable lower bound the energy gap, we use We find where we omitted non-negative summands. Now consider the following quantity, which will bound the individual terms in the previous equation, where the maximum is given by the smallest non-zero eigenvalue of . Hence and therefore we have the lower bound , where Injectivity may fail to hold in certain singular cases. The simplest example given by the family of GHZ-type states . As any local reduced density matrix is independent of φ , it is impossible to distinguish the members of that family based on local information alone. Indeed, in this example, the ground state space of Ĥ will be two-dimensional, spanned by |0,...,0〉 and |1,...,1〉. One may check that the gap analysis above continues to hold in the degenerate case (unlike the original in ref. 9 ), now certifying the overlap between ρ̂ and the ground-state space. This fact alone implies an exponential reduction in the number of unknown parameters. It is easy to see that the small remaining uncertainty about ρ̂ can be lifted in our example by measuring the 'string operator' , which has expectation value cos φ . Using, for example, the results of refs 38 , 39 , the method of this particular example immediately generalizes to any MPS with a two-fold degeneracy. Higher degeneracies may be treated by straightforward, but more tedious, methods. How to cite this article: Cramer, M. et al . Efficient quantum state tomography. Nat. Commun. 1:149 doi: 10.1038/ncomms1147 (2010).